High-efficiency motor neuron differentiation from human pluripotent stem cells and the function of Islet-1 Efficient derivation of large-scale motor neurons (MNs) from human pluripotent stem cells is central to the understanding of MN development, modelling of MN disorders in vitro and development of cell-replacement therapies. Here we develop a method for rapid (20 days) and highly efficient (~70%) differentiation of mature and functional MNs from human pluripotent stem cells by tightly modulating neural patterning temporally at a previously undefined primitive neural progenitor stage. This method also allows high-yield (>250%) MN production in chemically defined adherent cultures. Furthermore, we show that Islet-1 is essential for formation of mature and functional human MNs, but, unlike its mouse counterpart, does not regulate cell survival or suppress the V2a interneuron fate. Together, our discoveries improve the strategy for MN derivation, advance our understanding of human neural specification and MN development, and provide invaluable tools for human developmental studies, drug discovery and regenerative medicine. The derivation of human embryonic stem cells (hESCs) from blastocyst-stage embryos [1] and subsequent generation of induced pluripotent stem cells (iPSCs) from mouse and human somatic cells [2] , [3] , [4] , [5] offer unprecedented opportunities for scientific advancement, biomedical research and drug development. hESCs and human iPSCs (hiPSCs) can self-renew almost indefinitely in culture and have the remarkable potential to give rise to derivatives of all three embryonic germ layers. These human pluripotent stem cells therefore have been hailed as a possible means for treating degenerative, malignant, genetic diseases, or injuries due to inflammation, infection and trauma. Meanwhile, hESCs and hiPSCs are an invaluable research tool to study and model early human development (both normal and abnormal) and to understand fundamental biological questions such as cell proliferation, differentiation and cellular plasticity. Furthermore, they can serve as a platform for developing and testing new drugs. To fully realize the potential of hESCs and hiPSCs, the first and perhaps the most critical step is the directed differentiation of the cells to specific lineages with high efficiency and purity. Motor neurons (MNs) are a specialized class of neurons that reside in the spinal cord and project axons in organized and discrete patterns to muscles to control their activity. They are damaged in diseases such as spinal muscular atrophy and amyotrophic lateral sclerosis. Considerable progress has been made in the past decade in differentiating human pluripotent stem cells into MNs. A number of protocols have been developed, which utilize various themes including co-culture with stromal feeders (PA6 or MS5) [6] , embryoid body (EB) induction followed by neural rosette formation, neural patterning and neuronal maturation [7] , and neural progenitor induction from EBs followed by genetic programming using adenovirus-mediated gene delivery [8] . Despite these encouraging advances, limitations remain in the existing MN protocols that hamper the use of human pluripotent stem cells. For example, the differentiation procedures as they stand are tedious, time consuming (up to 2 months), requires genetic manipulations and repeated viral infections, and are of low efficiencies (10–40%) and yields [7] , [8] . Furthermore, the differentiation media and substrates contain undefined factors, animal feeder cells and/or animal products and are therefore not clinically compatible. Recently, several groups, including us, reported single-step procedures for neural induction of human pluripotent stem cells in adherent cultures [9] , [10] , [11] . Rapid (5–6 days) and high-efficiency (>80%) induction of PAX6 + neural progenitor cells (NPCs) can be attained by simultaneous inhibition of the bone morphogenetic protein (BMP) and Activin signalling pathways in hESCs and hiPSCs. The NPCs exhibit characteristics of early neuroepithelial cells of the anterior central nervous system, can form neural rosette structures and are thought to represent the most primitive hESC-derived neural progenitor stage isolated to date [9] . Because of the simplicity, flexibility, consistency and high efficiency, these methods offer powerful tools for subsequent derivation of subtypes of neural cells. In this study, based on high-efficiency neural induction, tightly controlled temporal modulation of neural patterning and fully optimized extracellular matrix (ECM) and medium conditions for neuronal maturation, we developed a method for rapid (~20 day), highly efficient (≈70%) and high-yield (>250%) production of mature and functional MNs from hESCs and hiPSCs in chemically defined adherent cultures. Thus, we have significantly improved the conditions for MN generation, which should facilitate the therapeutic applications of human MNs. Interestingly, we found that the motoneuron fate specification from human pluripotent stem cells requires exposure to neural patterning factors at a primitive stage (day 3) of neural differentiation, induced by compound C—a chemical inhibitor of Activin and BMP signalling [10] . These findings point to a primitive neural progenitor population that can adopt both the anterior and the posterior fate and arises much earlier during human neural specification than previously recognized. We applied our method to the molecular dissection of the mechanisms underlying human MN development and demonstrated for the first time that Islet-1 (ISL1) is required for formation of mature and functional human MNs from hESCs. Interestingly, unlike mouse ISL1, which, when deleted or reduced, leads to the loss of MNs and conversion to the V2a interneuron fate in mice [12] , [13] , [14] , depletion of human ISL1 did not cause cell death or V2a interneuron conversion, implying distinct regulatory mechanisms between humans and rodents in MN development. Therefore, our MN differentiation model also provides a powerful tool for studying the molecular programmes for both normal and abnormal human neural development. Neural induction under chemically defined conditions We recently developed a single-step method for neural induction of hESCs and hiPSCs in adherent cultures [10] . Our method is based on the use of a chemical compound—compound C—which targets multiple tumour growth factor-β superfamily receptors and consequently blocks both the Activin and BMP pathways in hESCs. We cultured H1 and H9 hESCs or hiPSC lines to confluency and subsequently differentiated the cells in compound C-containing medium [10] . This and other similar methods based on the principle of dual inhibition of BMP and Activin signalling led to the formation of PAX6 + NPCs within 5–6 days, with an efficiency of up to 90% (refs 9 , 10 , 11 ). In this study, we used the compound C-based neural induction method to explore new conditions for motoneuron generation from hESCs. As a first step towards attaining this goal, we made several modifications to the neural induction procedure. First, we cultured hESCs in the recently developed E8 medium [15] and on ECM substrates consisting of fibronectin, vitronectin and laminin, before compound C induction ( Fig. 1a,c ). The goal of these modifications was to substitute previously used chemically undefined components (mTeSR1 medium and Matrigel) to develop chemically defined conditions. Vitronectin and fibronectin were selected because of earlier documentations that they are capable of supporting the long-term self-renewal of human pluripotent stem cells [16] , [17] , while laminin reportedly enhances the proliferation and survival of NPCs [18] . In addition, we replaced chemically undefined knockout serum replacement with chemically defined N2 medium for neural induction. N2 medium is more commonly used for neural differentiation [19] , [20] . Under the new conditions, we found that compound C was also capable of inducing high-efficiency early neural differentiation in hESCs, as shown by the large percentage of PAX6 + NPCs (87.5±8.8%; n =6) (mean±s.d. ; see Methods ) 6 days after induction of differentiation ( Fig. 1b ). Expectedly, expression of markers for endoderm and mesoderm such as SOX17, T and GATA6 was largely undetected (<1%; n =6). Thus, we developed conditions for high-efficiency production of NPCs under chemically defined conditions. For the following experiments, we used both undefined (that is, mTeSR1 and Matrigel) and chemically defined condition (that is, E8 and fibronectin/vitronectin/laminin) to derive NPCs from hESCs and hiPSCs, with the latter condition more suited for clinically compatible derivation. 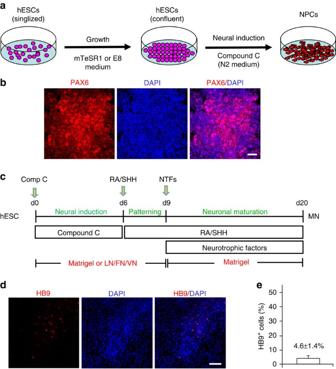Figure 1: Neural induction and MN differentiation from hESCs. (a) Schematic overview of neural induction of hESCs. See text for detail. (b) Immunofluorescence of PAX6 (red) in H1 hESCs induced to differentiate for 6 days with compound C (1 μM). Cell nuclei were stained with DAPI (4',6-diamidino-2-phenylindole; blue). Scale bar, 50 μm. (c) Diagram showing initial protocol used for MN induction from hESCs. Comp C denotes compound C. LN, FN and VN denote laminin, fibronectin and vitronectin, respectively. (d) Immunofluorescence of HB9 (red) in H1 hESCs after 20-day differentiation. Cells were induced to differentiate based on the MN procedure described inc, with Matrigel as the substrate for neuronal maturation. Cell nuclei were stained with DAPI (blue). Scale bar, 50 μm. (e) The percentage of HB9+cells of total differentiated cells (as indicated by DAPI). The bar represents the mean±s.d. (error bars) of six separate experiments. Figure 1: Neural induction and MN differentiation from hESCs. ( a ) Schematic overview of neural induction of hESCs. See text for detail. ( b ) Immunofluorescence of PAX6 (red) in H1 hESCs induced to differentiate for 6 days with compound C (1 μM). Cell nuclei were stained with DAPI (4',6-diamidino-2-phenylindole; blue). Scale bar, 50 μm. ( c ) Diagram showing initial protocol used for MN induction from hESCs. Comp C denotes compound C. LN, FN and VN denote laminin, fibronectin and vitronectin, respectively. ( d ) Immunofluorescence of HB9 (red) in H1 hESCs after 20-day differentiation. Cells were induced to differentiate based on the MN procedure described in c , with Matrigel as the substrate for neuronal maturation. Cell nuclei were stained with DAPI (blue). Scale bar, 50 μm. ( e ) The percentage of HB9 + cells of total differentiated cells (as indicated by DAPI). The bar represents the mean±s.d. (error bars) of six separate experiments. Full size image MN differentiation from NPCs The NPCs generated via dual inhibition of BMP and Activin signalling after the 6-day differentiation resemble the early neuroepithelial cells during human neural development [9] , leading us to examine whether they could be further induced to undergo terminal MN differentiation. We followed the developmental principles for neural development and applied a three-step strategy—neural induction, neural patterning and neuronal maturation—to MN differentiation from human pluripotent stem cells ( Fig. 1c ). Accordingly, we exposed the compound C-induced NPCs to retinoic acid (RA), a caudalizing factor, and sonic hedgehog (SHH), a ventralizing morphogen, to specify the ventral spinal fate [21] ( Fig. 1c ). After RA/SHH patterning, cells were re-plated on Matrigel and treated with neurotrophic factors, including brain-derived neurotrophic factor, cAMP, glial cell-derived neurotrophic factor and insulin-like growth factor-1 to induce neuronal maturation ( Fig. 1c ). Twenty days after differentiation was initiated, nuclear expression of the motoneuron marker HB9 was observed, suggesting formation of spinal MNs ( Fig. 1d ). However, quantification of HB9 + cells indicated that the differentiation efficiency was very low (4.6±1.4%; n =6; Fig. 1e ). In addition, when seeded as single cells on Matrigel for induction of maturation, the cells exhibited poor adhesion and were venerable to apoptosis, resulting in an extremely low survival rate at the end of the maturation process (1.5%±0.4; n =10). Instead, high-density plating of clustered cells on Matrigel was needed for sustained survival. Thus, this procedure ( Fig. 1c ) produces a low efficiency of motoneuron differentiation and is limited to high-density aggregate cultures for neuronal differentiation and maturation. Temporal control of patterning impacts MN differentiation The weak response of cells to RA and SHH patterning was surprising. During mouse neural development, establishment of MN identity is controlled temporally and spatially by the morphogenic activities of RA and SHH [21] . After being generated by retinaldehyde dehydrogenase in the presomitic mesoderm at E7.5, RA is released and travels to adjacent posterior neuroectoderm in the caudal neural plate, where it induces differentiation of progenitor MNs by activating various homeobox genes [22] . RA-mediated caudal progenitor MN patterning is followed by dorsoventral patterning induced by SHH [21] . Together, these earlier findings led us to hypothesize that the weak MN specification might be improved with more precise temporal modulation of the patterning factors during neural induction. To test this, we conducted time-course analysis of the expression pattern of neuroepithelial markers (PAX6, SOX1 and ZIC1) and pluripotency markers (OCT-4 and NANOG), leading us to identify three potential phases of neural induction. In the first phase (day 0–1 after neural induction), the protein levels of PAX6/SOX1/ZIC1 or OCT-4/NANOG, as shown by western blotting analysis, were altered only moderately ( Fig. 2a,b and Supplementary Fig. 5 ). In the second phase (day 1–3), both the neural progenitor and pluripotency markers underwent rapid changes in protein levels, increasing (for PAX6, SOX1 and ZIC1) or decreasing (for OCT-4 and NANOG) dramatically ( Fig. 2a,b and Supplementary Fig. 5 ). In contrast, after day 3, the level of PAX6, SOX1 and ZIC1 increased moderately ( Fig. 2a,b and Supplementary Fig. 5 ). The level of OCT-4 and NANOG further declined and was nearly undetectable at day 6 of neural induction ( Fig. 2a,b and Supplementary Fig. 5 ). 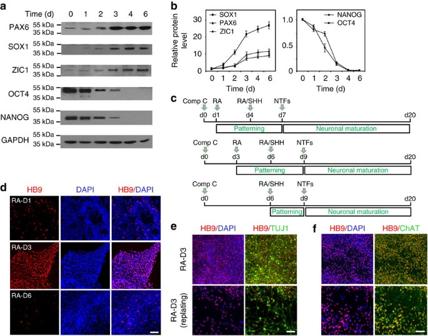Figure 2: Rapid and high-efficiency MN differentiation via temporal modulation of RA/SHH patterning. (a) Western blotting of neural progenitor and pluripotency markers at various time points after neural induction of H1 hESCs with compound C. A typical experiment from five separate experiments is shown. GAPDH was a loading control. (b) Quantification of protein levels of the neural progenitor (left) and pluripotency markers (right). The experiments were as described ina. Y-axis represents relative intensities (measured with Image J) with values normalized to the signal (=1) before neural induction (day 0). Each bar represents mean±s.d. (error bars). Five separate experiments were analysed. (c) Schematic overview of three strategies for MN differentiation used in our study. A key variable is the timing of RA-induced patterning during the course of differentiation. Specifically, RA was added to cells at day 1, day 3 and day 6 during neural induction with compound C. Compound C was applied for neural induction for 6 days for all three strategies (day 0–day 6). (d) Immunofluorescence of HB9 (red) in H1 hESCs after 20-day differentiation. MN differentiation was induced based on the schemes described inc. Cell nuclei were stained with DAPI (4',6-diamidino-2-phenylindole; blue). RA-D1, RA-D3 and RA-D6 denote the time of initiation of RA patterning (at day 1, day 3 and day 6, respectively). (e) Top: merged fluorescence images of HB9/DAPI (left) and HB9/TUJ1 (right) staining of differentiated cells (at day 20 with patterning initiated at day 3). Bottom: merged fluorescence images of HB9/DAPI (left) and HB9/TUJ1 (right) staining of differentiated cells replated at a low density for 3–4 days after 20-day differentiation (denoted as ‘replating’). (f) Top: merged fluorescence images of HB9/DAPI (left) and HB9/ChAT (right) staining of differentiated cells (at day 20 with patterning initiated at day 3). Bottom: merged fluorescence images of HB9/DAPI (left) and HB9/ChAT (right) staining of differentiated cells replated at a low density for 3–4 days after 20-day differentiation. All scale bars, 50 μm. Figure 2: Rapid and high-efficiency MN differentiation via temporal modulation of RA/SHH patterning. ( a ) Western blotting of neural progenitor and pluripotency markers at various time points after neural induction of H1 hESCs with compound C. A typical experiment from five separate experiments is shown. GAPDH was a loading control. ( b ) Quantification of protein levels of the neural progenitor (left) and pluripotency markers (right). The experiments were as described in a . Y-axis represents relative intensities (measured with Image J) with values normalized to the signal (=1) before neural induction (day 0). Each bar represents mean±s.d. (error bars). Five separate experiments were analysed. ( c ) Schematic overview of three strategies for MN differentiation used in our study. A key variable is the timing of RA-induced patterning during the course of differentiation. Specifically, RA was added to cells at day 1, day 3 and day 6 during neural induction with compound C. Compound C was applied for neural induction for 6 days for all three strategies (day 0–day 6). ( d ) Immunofluorescence of HB9 (red) in H1 hESCs after 20-day differentiation. MN differentiation was induced based on the schemes described in c . Cell nuclei were stained with DAPI (4',6-diamidino-2-phenylindole; blue). RA-D1, RA-D3 and RA-D6 denote the time of initiation of RA patterning (at day 1, day 3 and day 6, respectively). ( e ) Top: merged fluorescence images of HB9/DAPI (left) and HB9/TUJ1 (right) staining of differentiated cells (at day 20 with patterning initiated at day 3). Bottom: merged fluorescence images of HB9/DAPI (left) and HB9/TUJ1 (right) staining of differentiated cells replated at a low density for 3–4 days after 20-day differentiation (denoted as ‘replating’). ( f ) Top: merged fluorescence images of HB9/DAPI (left) and HB9/ChAT (right) staining of differentiated cells (at day 20 with patterning initiated at day 3). Bottom: merged fluorescence images of HB9/DAPI (left) and HB9/ChAT (right) staining of differentiated cells replated at a low density for 3–4 days after 20-day differentiation. All scale bars, 50 μm. Full size image Consistent with the results of western blotting, immunofluorescence of PAX6 and SOX1 also revealed drastic increases in the number of PAX6 + , SOX1 + and PAX6 + /SOX1 + cells from day 1 to day 3 after neural induction ( Supplementary Fig. 1a ). Furthermore, the number of PAX6 + , SOX1 + and PAX6 + /SOX1 + cells continued to increase at day 6 ( Supplementary Fig. 1a ). Moreover, dual immunofluorescence labelling of PAX6 and OCT-4 demonstrated a large population of PAX6 + /OCT-4 + cells at day 3 of neural induction (65.1±3.8%; n =5; Supplementary Fig. 1b ), although the overall levels of PAX6 and OCT-4 proteins at day 3 of neural induction were lower than that at day 1 (for OCT-4) or day 6 (for PAX6). In contrast, such PAX6 + /OCT-4 + cell populations were largely absent at day 1 and day 6 (<1%; n =5). As RA and SHH addition at the late-phase neural induction (that is, day 6) led to poor motoneuron differentiation ( Fig. 1c–e ), we tested the temporal effect of introducing RA at the first phase (that is, at day 1) and the second phase (that is, at day 3) of neural induction (with a 6-day compound C treatment) and compared with RA stimulation at day 6 ( Fig. 2c ). Remarkably, initiation of RA treatment at day 3 followed by subsequent neuronal maturation led to a high percentage of HB9 + cells from H1 hESCs (66.3±10.9%; n =10; Fig. 2d ), whereas a parallel treatment of RA initiated at day 1 produced a much smaller number of HB9 + cells (9.0±5.7%; n =10; Fig. 2d ). The HB9 + cells produced with RA addition at day 3 also expressed TUJ1, a neuronal marker ( Fig. 2e and Supplementary Fig. 2a ), choline acetyltransferease (ChAT) that catalyses synthesis of acetylcholine, a neuron transmitter and is found exclusively in the MNs in the ventral spinal cord [23] ( Fig. 2f ), and SMI-32, a non-phosphorylated neurofilament marker that stains MNs in the spinal cord [24] , [25] ( Supplementary Fig. 2b ). To minimize the potential complications in examination of neuronal morphology and MN quantifications caused by high-density cultures, we replated MNs produced with RA treatment initiated at day 3 at a lower cell density. We analysed the efficiency of differentiation 3–4 days after replating and detected a similar high percentage of HB9 + cells (69.5±11.2%; n =6; Fig. 2e–f and Supplementary Fig. 2c ; denoted as ‘replating’) that were also positive for TUJ1, ChAT and SMI-32 ( Fig. 2e,f and Supplementary Fig. 2d ). In addition, we observed dramatic increases in the mRNA level of HB9 , ChAT, Nkx6.1 , NeuroD1 and HoxC4 in cells with patterning initiated at day 3 versus those at day 6, further verifying motoneuron specification ( Supplementary Fig. 2e ). Importantly, initiation of RA treatment at day 3 followed by subsequent neuronal maturation also produced a high percentage of HB9 + cells (60.1±9.5%; n =8) from H9 hESCs, suggesting conserved responses in hESCs. Next, we determined whether the hESC-derived MNs were functional using established assays [8] , [26] , [27] , [28] . First, the cells were capable of extending long projections, suggesting neuronal maturation ( Fig. 3a ). Second, co-localization of Map2 + neurites with synapsin I and TUJ1 + neurites with synaptic vesicle protein 2 was detected, indicating synaptic activities ( Fig. 3b,c ; synapsin I and synaptic vesicle protein 2 are synaptic markers). Map2 immunoreactivity is present in both axons and dendrites of spinal MNs [29] , [30] . In addition, when the neurons were co-cultured with differentiated myotubes from mouse C2C12 cells, co-localization of acetylcholine receptors with ChAT + neurites was observed ( Fig. 3d ), suggesting formation of neuromuscular junctions. Finally, we used whole-cell patch clamp recordings to determine the electrophysiological properties of the MNs produced. We found that 69% of the cells ( n =32) were electrophysiologically active, as defined by their ability to elicit short-lasting action potentials in response to depolarizing current injection in current–clamp recordings ( Fig. 3e,f ). These action potentials were blocked by the voltage-gated sodium channel blocker tetrodotoxin (TTX, 1 μM), suggesting that they were functional action potentials ( Fig. 3g ). Next, we recorded transient sodium currents from these cells. Using voltage–clamp recording techniques, sodium currents were evoked by applying depolarizing voltage steps. Under these conditions, a strong transient inward current was evoked and this current was completely blocked by TTX, indicating that this indeed was a sodium current characteristic of functional neurons ( Fig. 3h ). In multiple neurons, we were able to evoke tonic action potential discharge with small depolarization of the membrane potential ( Fig. 3i ). Thus, stage-specific neural patterning during neural induction of hESCs leads to high-efficiency derivation of mature and functional MNs from hESCs. 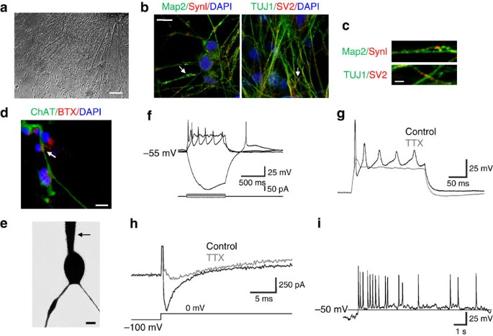Figure 3: MNs derived from hESCs are mature and electrophysiologically active. (a) Phase-contrast image of neurons extending long projections. Scale bar, 50 μm. (b) Confocal fluorescence microscopy images showing Map2, synapsin I (SynI) and DAPI (4',6-diamidino-2-phenylindole; merged, left) and TUJ1, synaptic vesicle protein 2 (SV2) and DAPI (merged, right) staining in cells after 20-day differentiation from H1 hESCs. The arrows point to synapsin and SV2-positive synaptic structures. Scale bar, 10 μm. (c) Corresponding enlarged images fromb. Scale bar, 5 μm. (d) MNs, stained with ChAT antibody (green), form neuromuscular junctions, labelled with bungarotoxin (BTX, red), when cultured on myotubes. Cell nuclei were stained with DAPI (blue). Arrow shows co-localization of ChAT-positive neurites with BTX. Myotubes were differentiated from mouse C2C12 cells. Scale bar, 20 μm. (e) Image of a neuron filled with fluorescent dye (Alexa594) under electrophysiological examination, with the patch pipette indicated by the arrow. Scale bar, 10 μm. (f) Representative voltage traces showing response to current injections. Note the action potentials evoked by depolarizing current injections. (g) In same cell asf, depolarizing current step evokes multiple action potentials that are completely blocked by TTX (1 μM). (h) Using voltage clamp recording technique, a transient inward current is evoked by depolarizing current step. This inward current is completely attenuated by TTX, indicating this response is a sodium current. (i) In some cells, small depolarization of the membrane potential could evoke tonic discharge of action potentials. Figure 3: MNs derived from hESCs are mature and electrophysiologically active. ( a ) Phase-contrast image of neurons extending long projections. Scale bar, 50 μm. ( b ) Confocal fluorescence microscopy images showing Map2, synapsin I (SynI) and DAPI (4',6-diamidino-2-phenylindole; merged, left) and TUJ1, synaptic vesicle protein 2 (SV2) and DAPI (merged, right) staining in cells after 20-day differentiation from H1 hESCs. The arrows point to synapsin and SV2-positive synaptic structures. Scale bar, 10 μm. ( c ) Corresponding enlarged images from b . Scale bar, 5 μm. ( d ) MNs, stained with ChAT antibody (green), form neuromuscular junctions, labelled with bungarotoxin (BTX, red), when cultured on myotubes. Cell nuclei were stained with DAPI (blue). Arrow shows co-localization of ChAT-positive neurites with BTX. Myotubes were differentiated from mouse C2C12 cells. Scale bar, 20 μm. ( e ) Image of a neuron filled with fluorescent dye (Alexa594) under electrophysiological examination, with the patch pipette indicated by the arrow. Scale bar, 10 μm. ( f ) Representative voltage traces showing response to current injections. Note the action potentials evoked by depolarizing current injections. ( g ) In same cell as f , depolarizing current step evokes multiple action potentials that are completely blocked by TTX (1 μM). ( h ) Using voltage clamp recording technique, a transient inward current is evoked by depolarizing current step. This inward current is completely attenuated by TTX, indicating this response is a sodium current. ( i ) In some cells, small depolarization of the membrane potential could evoke tonic discharge of action potentials. Full size image A primitive NPC stage between hESCs and anterior NPCs Why does initiation of patterning at day 3 of neural induction lead to high-efficiency MN differentiation while such treatment causes cells with 6-day compound C induction to respond poorly? We first asked whether there were major changes in expression of key RA signalling components in hESCs after neural induction. Experiments with real-time PCR analysis revealed very small differences in the levels of RA receptors ( RARA, RARB and RARG ) and retinoid X receptors ( RXRA , RXRB and RXRG , which heterodimerize with RA receptors) at day 3 and day 6 ( Table 1 ). We also examined the levels of NCOA1 ( SRC-1 ), NCOA2 ( SRC-2 ), NCOA3 ( SRC-3 ), EP300 ( p300 ), KAT2B ( pCAF ) and CREBBP ( CBP ), co-activators of nuclear receptors that promote transcription in conjunction with nuclear receptors. As shown in Table 1 , expression of NCOA1 , EP300 and CREBBP was similar in cells at day 3 and day 6 of compound C induction, while NCOA2 , NCOA3 and KAT2B were upregulated at day 6. These results strongly suggest that the differential effects of RA patterning were not due to alterations of key RA signalling components. Table 1 Expression of RA signalling, forebrain and hindbrain genes during neural induction. Full size table We next explored the possibility that the late-stage NPCs (that is, at day 6 of neural induction) respond poorly to patterning factors because they might be more committed to the anterior neural fate than previously recognized and thus possess declined caudalization potential. This notion was also supported by a recent report that prolonged dual inhibition (for ⩾ 6 days) of Activin and BMP signalling in hESCs with small molecules induces differentiation of cell characteristic of the anterior neural ectoderm [11] . To test this possibility, we assessed the expression pattern of markers for forebrain/hindbrain lineage restrictions during neural induction of hESCs (that is, 0, 1, 3 and 6 days after compound C treatment). The neural markers were selected largely in correlation with earlier studies [11] . Of the 20 forebrain-specific genes examined, 17 genes ( RAX , OTX1 , OTX2 , NR2F1 , NR2F2 , POU3F1 , POU3F2 , HESX1 , FEZF1 , LHX2 , ZEB2 , EMX2 , FEZF2 , CNTNAP2 , SIX3 , ARX and WNT7B ) were found to upregulate significantly (>2-fold) ( P <0.01; analysis of variance), with 12 genes exhibiting strong upregulation (>10-fold) at day 6 of neural induction versus day 0 ( Table 1 ). Importantly, 15 forebrain-specific genes showed significantly higher expression at day 6 of neural induction than day 3 ( Table 1 ). In contrast, of the 19 hindbrain-specific genes examined, only 4 genes exhibited more than 2-fold upregulation at day 6 of neural induction versus day 0, with none exceeding 10-fold ( Table 1 ). In addition, nine hindbrain-specific genes ( CEP290 , EGFL7 , CACNA1A , RORA , MTPN , HSPA5 , ULK1 , HES3 and GNPAT ) were continuously suppressed from day 3 to day 6 of compound C induction, whereas two genes ( GBX2 and MAFB ) were downregulated at day 1 and remained suppressed throughout neural induction ( Table 1 ). Taken together, our results suggest that prolonged compound C treatment for 6 days promotes anterior neuroectoderm fate specification of hESCs, in keeping with previous findings [11] . The lineage bias towards the anterior fate provides mechanistic explanations for the poor responses of the cells with 6-day compound C induction to the patterning stimulation. Furthermore, our findings indicate that a more primitive neural progenitor stage may arise as early as day 3 after neural induction from human pluripotent stem cells. This potential primitive NPC population possesses the potential to be readily processed to adopt the posterior neural fate in the presence of patterning factors, and can also become anterior NPCs with prolonged compound C treatment. High-yield MN maturation under chemically defined conditions Having identified the neural patterning conditions allowing for high-efficiency MN differentiation, we next addressed another issue associated with MN derivation from hESCs—poor cell survival during neuronal maturation. As described earlier in this study, when plated on Matrigel as single cells for neuronal maturation induction, the neural cells exhibited a low survival rate ( Figs 1c and 4a,b , and Table 2 ). Furthermore, the Matrigel matrix consists of undefined ECM components and growth factors and is potentially xenogeneic. These limitations could hamper the use of the MN differentiation protocols for research and clinical efforts such as clonal isolation, drug screening and cell therapies. We therefore replaced Matrigel with chemically defined ECM molecules. Despite the report that laminin can support long-term expansion of neural progenitors [18] , when used alone it failed to support the survival of single hESC-derived neural cells (1.4±0.3%; n =6; Table 2 ). We then tested other ECM molecules, including Collagen I (COLI), IV (COLIV) and fibronectin, which, when used individually, also led to similar low survival rates (<2%; n =6; Table 2 ). Interestingly, two of these ECM substrates in combination slightly improved cell survival (<5%; n =6), whereas the use of three substrates combined caused much stronger effects ( Fig. 4b ). Furthermore, an optimal effect (91±8%; n =6) was observed when laminin, COLI, COLIV and fibronectin were combined ( Fig. 4a,b and Table 2 ). When cultured on substrates consisting of these four ECM molecules, MNs could be maintained for at least a month with no apparent changes in cell survival and activities. We also calculated the yield of MN production as the percentage of HB9 + cells in relation to the initial number of hESCs plated. Using this calculation we found that the improved method using combined four matrix proteins produced a motoneuron yield of 252.4±30.3% ( n =6) from hESCs ( Fig. 4c ). Thus, by developing new substrate conditions, we obtained high-yield MN maturation and long-term MN survival under chemically defined conditions. 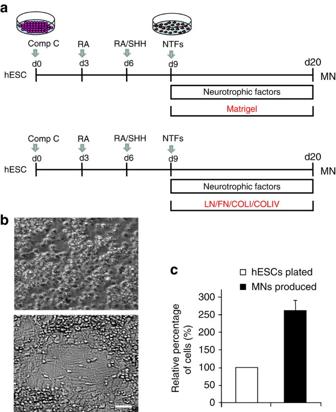Figure 4: Maturation of MNs under chemically defined conditions. (a) Schematic overview showing the ECM substrates used to induce maturation of MNs derived from hESCs. Laminin (LN), fibronectin (FN), Collagen I (COLI) and Collagen IV (COLIV) in combination (bottom) can replace Matrigel (top) for induction of neuronal maturation. (b) Representative phase-contrast images of cells collected 6 days after initiation of neuronal maturation. Cells plated as single cells on Matrigel showed massive cell death (top), while cells plated on the matrix mix (LN/FN/COLI/COLIV) continued to differentiate with minimal cell death (bottom). Scale bar, 50 μm. (c) The yield of MN production calculated as the percentage of HB9+cells after 20-day differentiation in relation to the initial number of hESCs plated (100%). MNs were derived from hESCs under conditions described ina, with LN/FN/COLI/COLIV as the substrate. The value is mean±s.d. of six independent experiments. Figure 4: Maturation of MNs under chemically defined conditions. ( a ) Schematic overview showing the ECM substrates used to induce maturation of MNs derived from hESCs. Laminin (LN), fibronectin (FN), Collagen I (COLI) and Collagen IV (COLIV) in combination (bottom) can replace Matrigel (top) for induction of neuronal maturation. ( b ) Representative phase-contrast images of cells collected 6 days after initiation of neuronal maturation. Cells plated as single cells on Matrigel showed massive cell death (top), while cells plated on the matrix mix (LN/FN/COLI/COLIV) continued to differentiate with minimal cell death (bottom). Scale bar, 50 μm. ( c ) The yield of MN production calculated as the percentage of HB9 + cells after 20-day differentiation in relation to the initial number of hESCs plated (100%). MNs were derived from hESCs under conditions described in a , with LN/FN/COLI/COLIV as the substrate. The value is mean±s.d. of six independent experiments. Full size image Table 2 Survival rates of cells under various matrix conditions. Full size table It was previously reported that Matrigel contains ECM molecules, including laminin, COLIV, enactin and heparan sulphate proteoglycan, but has only small amounts of fibronectin and COLI (refs 31 , 32 ). We therefore asked whether the addition of fibronectin and COLI to Matrigel could improve Matrigel’s ability to support cell survival. Interestingly, the combined use of Matrigel/fibronectin or Matrigel/fibronectin/COLI only moderately increased the rates of cell survival (from 1.2±0.3% with Matrigel alone, to 3.5±1.2% and 10.2±3.6% with Matrigel/fibronectin and Matrigel/fibronectin/COLI, respectively; n =6). Thus, the supply of fibronectin and COLI to Matrigel failed to mimic the effect of the chemically defined substrates composed of laminin, COLI, COLIV and fibronectin. The contributing factor(s) to the poor ability of Matrigel to support survival of dissociated differentiating cells remain to be defined. A recent study showed that in addition to ECM molecules, Matrigel contains >1,200 unique proteins, including many directly related to the binding and signalling of growth factors [33] . High-efficiency MN differentiation from hiPSCs Human iPSCs can be induced from somatic cells with defined transcription factors and exhibit similar properties to hESCs when fully reprogrammed [34] . As demonstrated earlier, our method was highly effective for motoneuron induction from hESCs, leading us to ask whether it could also be applied to hiPSCs. We used three previously established hiPSC lines—MMW2, RND5 and ID28. MMW2 and RND5 lines were derived by the use of lentivirus-mediated gene delivery [10] , [35] , while the ID28 hiPSC line was generated using an integration-free reprogramming approach [36] . When cultured under self-renewal conditions, these hiPSC lines all exhibited typical pluripotent stem cell morphologies and expressed pluripotent markers OCT-4 and NANOG ( Supplementary Fig. 3a ) [10] , [35] , [36] . When subjected to the motoneuron differentiation method developed for hESCs, hiPSCs exhibited a range of efficiencies. Both the RND5 and ID28 cells responded well to compound C induction by forming 70–80% PAX6 + cells, whereas the MMW2 cells only differentiated to <20% PAX6 + cells ( n =5; Supplementary Fig. 3b ). Furthermore, although the RND5 cells exhibited a high survival rate (~80%) after cultivation under the neural patterning and neuronal maturation conditions, they only differentiated into ~30% TUJ1 + cells and <2% HB9 + cells ( n =5). In contrast, the ID28 hiPSC line differentiated into a high percentage of HB9 + TUJ1 + cells (51.6%±5.7; n =6) that were also positive for SMI32 after 18-day differentiation, with a high yield of differentiation (352.1± 41.5%, in relation to the initial number of ID28 cells plated; n =6; Supplementary Fig. 3c ). Interestingly, unlike hESCs, which had sustained HB9 protein expression from day 17 after differentiation, the ID28 hiPSC line showed transient HB9 expression, which emerged at day 15, peaked at day 18, but decreased at day 20 (to 21.2±5.1% of HB9 + cells; n =6; Supplementary Fig. 3c ). The hiPSC-derived MNs were mature and functional, as evidenced by their ability to develop mature synapse ( Supplementary Fig. 3d ), form neuromuscular junctions ( Supplementary Fig. 3e ), and become electrophysiologically active ( Supplementary Fig. 3f–i ). Thus, our method is effective for hiPSC differentiation and can therefore be broadly applied for MN derivation from human pluripotent stem cells. The cell-line related variability in motoneuron differentiation efficiencies for NPCs and hiPSCs is consistent with earlier reports [28] , [37] . The factors that contribute to the discrepancies in MN differentiation between hESCs and hiPSCs remain to be defined. ISL1 is a key regulator of human motoneuron development The MN-directed differentiation method is based on adherent cultures, produces MN populations with high purity and efficiency, recapitulates MN development in real time and can be readily manipulated genetically. Thus, we argued that in addition to its therapeutic values, this method could be used as a dynamic model for dissecting the molecular programmes underlying human motoneuron fate determination quantitatively. To test this possibility we assessed the role of ISL1 in human MN differentiation. ISL1, a member of the LIM/homeodomain family of transcription factors, is expressed in all MN subtypes and essential for MN generation in mice and Xenopus . ISL1 is immediately expressed in prospective MNs when they exit cell cycle, and ISL1 deletion or hypomorphic mutations lead to the loss of spinal MN populations and conversion to Chx10-positive V2a interneurons in mice [12] , [13] , [14] , suggesting that ISL1 functions to maintain MN identity against interneurons. Islet is also required for axon projection and neurotransmitter expression of MNs in Drosophila [38] and zebrafish [39] . Despite these findings, ISL1 function has not been defined in human-based neural development models. We first assessed the expression pattern of ISL1. When stimulated by RA at day 3 and subsequently induced to undergo neuronal maturation, hESCs began to express ISL1 protein at day 13 after differentiation. The expression of ISL1 protein peaked at day 15, when 76.1±5.8% of cells were positive ( n =6; Fig. 5a,b ). The high percentage of ISL1 + cells was further verified through analysis of differentiated cells replated at a lower density (78.3±3.5%; n =5; Fig. 5c ). As expected, cells with RA exposure at day 1 and day 6 exhibited low levels of ISL1 (10.9±3.4% and 7.2±1.4%, respectively; n =6; Fig. 5a,b ), consistent with the low-efficiency MN differentiation in the long term. In addition, the ID 28 hiPSCs exhibited a high level of ISL1 at day 14 after MN differentiation (65.4±5.1%; n =6), while the RND5 hiPSCs showed a much lower level (4.8%±1.1%; n =6; Supplementary Fig. 4a ). Thus, stage-specific neural patterning is essential for induction of ISL1 expression, which precedes the expression of HB9 during motoneuron development of human pluripotent stem cells. 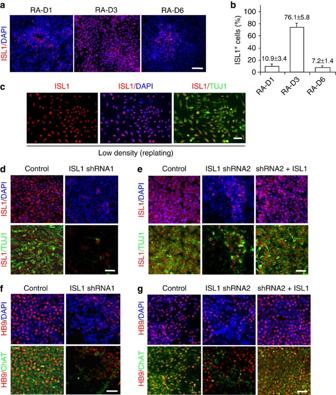Figure 5: ISL1 is a critical regulator of human motoneuron development. (a) Immunofluorescence of ISL1 (red) in cells after 15-day differentiation from H1 hESCs. Cell nuclei were stained with DAPI (4',6-diamidino-2-phenylindole; blue). RA-D1, RA-D3 and RA-D6 denote the time of initiation of RA patterning (at day 1, day 3 and day 6, respectively). (b) Percentage of ISL1-positive cells under conditions described ina. Each bar represents mean±s.d. (error bars) of six experiments. (c) Fluorescence images of ISL1 (left), ISL1/DAPI (middle) and ISL1/ TUJ1 (right) staining in differentiated cells replated at a low density for 3 days after 15-day differentiation. (d) Fluorescence images of differentiated hESCs with NT shRNA (‘Control’, left) or with ISL1 shRNA-1 (‘ISL shRNA-1’, right) stained with antibodies against ISL1 (red) and TUJ1 (green) after 15-day differentiation (with patterning initiated at day 3). Cell nuclei were stained with DAPI (blue). (e) Fluorescence images of differentiated hESCs with NT shRNA (‘Control’, left), ISL1 shRNA-2 (‘ISL shRNA-2’, middle) and ISL1 shRNA-2 with ectopic ISL1 expression (‘shRNA-2+ISL1’, right) stained with antibodies against ISL1 (red) and TUJ1 (green) after 15-day differentiation (with patterning initiated at day 3). Cell nuclei were stained with DAPI (blue). (f) Fluorescence images of differentiated hESCs with NT shRNA (left) or with ISL1 shRNA (right) stained with antibodies against HB9 (red) and ChAT (green) after 20-day differentiation. Cell nuclei were stained with DAPI (blue). (g) Fluorescence images of differentiated hESCs with NT shRNA (left), ISL1 shRNA-2 (middle) and ISL1 shRNA-2, with ectopic ISL1 expression (right) stained with antibodies against HB9 (red) and ChAT (green) after 20-day differentiation (with patterning initiated at day 3). Cell nuclei were stained with DAPI (blue). All scale bars, 50 μm. Figure 5: ISL1 is a critical regulator of human motoneuron development. ( a ) Immunofluorescence of ISL1 (red) in cells after 15-day differentiation from H1 hESCs. Cell nuclei were stained with DAPI (4',6-diamidino-2-phenylindole; blue). RA-D1, RA-D3 and RA-D6 denote the time of initiation of RA patterning (at day 1, day 3 and day 6, respectively). ( b ) Percentage of ISL1-positive cells under conditions described in a . Each bar represents mean±s.d. (error bars) of six experiments. ( c ) Fluorescence images of ISL1 (left), ISL1/DAPI (middle) and ISL1/ TUJ1 (right) staining in differentiated cells replated at a low density for 3 days after 15-day differentiation. ( d ) Fluorescence images of differentiated hESCs with NT shRNA (‘Control’, left) or with ISL1 shRNA-1 (‘ISL shRNA-1’, right) stained with antibodies against ISL1 (red) and TUJ1 (green) after 15-day differentiation (with patterning initiated at day 3). Cell nuclei were stained with DAPI (blue). ( e ) Fluorescence images of differentiated hESCs with NT shRNA (‘Control’, left), ISL1 shRNA-2 (‘ISL shRNA-2’, middle) and ISL1 shRNA-2 with ectopic ISL1 expression (‘shRNA-2+ISL1’, right) stained with antibodies against ISL1 (red) and TUJ1 (green) after 15-day differentiation (with patterning initiated at day 3). Cell nuclei were stained with DAPI (blue). ( f ) Fluorescence images of differentiated hESCs with NT shRNA (left) or with ISL1 shRNA (right) stained with antibodies against HB9 (red) and ChAT (green) after 20-day differentiation. Cell nuclei were stained with DAPI (blue). ( g ) Fluorescence images of differentiated hESCs with NT shRNA (left), ISL1 shRNA-2 (middle) and ISL1 shRNA-2, with ectopic ISL1 expression (right) stained with antibodies against HB9 (red) and ChAT (green) after 20-day differentiation (with patterning initiated at day 3). Cell nuclei were stained with DAPI (blue). All scale bars, 50 μm. Full size image Next, we exploited our human MN differentiation model to study the function of ISL1 in human MN development. We screened a set of small hairpin RNAs (shRNAs) designed to target ISL1 by applying lentivirus-mediated knockdown in hESCs before the induction of neuronal maturation, which led us to identify two shRNAs (denoted as shRNA-1 and shRNA-2, respectively) that effectively reduced the mRNA level of ISL1 and the number of ISL1-positive cells ( Fig. 5d,e and Supplementary Fig. 4b,c ). ISL1 depletion did not induce cell death during differentiation (1.8±0.8% and 3.5±1.4% cell death for control and depleted cells, respectively; n =4), but markedly reduced the mRNA levels of HB9 and (to a greater extent) ChAT ( Supplementary Fig. 4b ). ISL1 depletion also significantly decreased the percentage of TUJ1 + cells at day 15 and HB9 + cells at the end of MN differentiation (that is, at day 20; Fig. 5d–g and Supplementary Fig. 4c ). It also reduced ChAT immunofluorescence signals ( Fig. 5f,g ). In addition, when co-cultured with differentiated C2C12 cells, ISL1-depleted cells failed to form neuromuscular junctions ( Supplementary Fig. 4d ). Thus, ISL1 is essential for induction of mature and functional MNs. Interestingly, ISL ectopic expression appeared insufficient to further increase the number of HB9 + cells after MN differentiation, producing 63.8±8.5% HB9 + cells ( n =5). To verify the specificity of ISL1 depletion, we ectopically expressed wild-type human ISL1 in differentiating hESCs with ISL1 depleted. We used shRNA-2, which targets 3′-untranslated region of ISL1 and thus specifically depletes endogenous ISL1, not ectopic ISL1. The endogenous gene products were depleted while the exogenously expressed mRNAs devoid of the 3′-untranslated region were resistant ( Supplementary Fig. 4b ). The ectopic expression of wild-type ISL1 largely rescued the defects in HB9, TUJ1 and ChAT caused by ISL1 depletion ( Fig. 5e,f and Supplementary Fig. 4b,c ). Finally, we examined whether ISL1 depletion during human MN differentiation also converts the cell identity to V2a interneurons, as reported for mouse ISL1 deletion and hypomorphic mutations [12] , [13] , [14] . We depleted ISL1 in hESCs using shRNA-1 and shRNA-2, which effectively reduced the level of ISL1 (at day 15) and HB9 mRNA (at day 20) after induction of differentiation ( Supplementary Fig. 4e,f ). ISL1 depletion did not significantly increase the mRNA level of Chx10 (a marker for V2a interneurons; Supplementary Fig. 4e,f ) or the number of Chx10-positive cells. Together, our experiments provide the first demonstration of ISL1 as a critical regulator of human motoneuron development. They also suggest that ISL1 controls human MN differentiation through distinct regulatory mechanisms from mouse ISL1. Developing conditions for rapid, efficient and high-yield derivation of MNs from human pluripotent stem cells is essential for neural developmental studies, drug screening and cell-replacement therapies. Several methods have been developed to differentiate MNs from hESCs or hiPSCs, but limitations still remain in these procedures. For instance, the protocols that use EB induction followed by RA/SHH-induced neural patterning and neuronal maturation are tedious, requiring up to 2 months to produce functional MNs, with relatively low efficiency (10–40%) [7] . More recently, a directed programming approach, based on adenoviral gene delivery of three MN-specific transcription factors Ngn2, ISL1 and Lhx3, can produce mature MNs from hESC/hiPSC-derived NPCs in 11 days (21 days from hESCs/hiPSCs) and leads to an efficiency of ~60% [8] . Notably, this protocol requires genetic manipulations and repeated high-titre viral infections, with the rate of cell survival and the yield of MN differentiation undetermined. Instead, our method exploits simple adherent cultures, is free from genetic manipulations, produces high yields (>250%) of mature and functional MNs from hESCs/hiPSCs within 20 days and is highly efficient (up to 70%). Furthermore, we have developed chemically defined medium and substrate conditions throughout neural induction, neural patterning, MN maturation, cultivation and maintenance ( Fig. 6a ). As such, our method has markedly improved the derivation of MNs from human pluripotent stem cells and is well suited for rapid, large-scale MN production under xeno-free and therapy-compatible conditions. 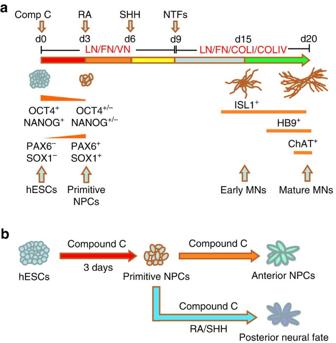Figure 6: Summary of the MN differentiation model and the stages of neural differentiation. (a) hESCs undergoing neural induction begin to express high levels of NPC markers, including PAX6 and SOX1 at day 3, while markedly downregulating the pluripotency markers such as OCT-4 and NANOG (albeit retaining some degree of expression). Thus, the cells at day 3 might represent a population of primitive NPCs that can be induced to become anterior NPCs and also possesses the potential to differentiate posteriorly. With neural patterning initiated at day 3 after neural induction, the early MN marker ISL1 can be seen at day 13 after hESC differentiation, while mature MN markers including HB9 and ChAT are expressed after 17-day differentiation. (b) Our results point to a previously unidentified primitive stage of neural progenitors that is intermediate between pluripotent hESCs and anterior NPCs. This population of potential primitive NPCs can be induced to become anterior NPCs in the absence of patterning factors, and also possesses the potential to differentiate along the posterior fate in the presence of patterning factors. Figure 6: Summary of the MN differentiation model and the stages of neural differentiation. ( a ) hESCs undergoing neural induction begin to express high levels of NPC markers, including PAX6 and SOX1 at day 3, while markedly downregulating the pluripotency markers such as OCT-4 and NANOG (albeit retaining some degree of expression). Thus, the cells at day 3 might represent a population of primitive NPCs that can be induced to become anterior NPCs and also possesses the potential to differentiate posteriorly. With neural patterning initiated at day 3 after neural induction, the early MN marker ISL1 can be seen at day 13 after hESC differentiation, while mature MN markers including HB9 and ChAT are expressed after 17-day differentiation. ( b ) Our results point to a previously unidentified primitive stage of neural progenitors that is intermediate between pluripotent hESCs and anterior NPCs. This population of potential primitive NPCs can be induced to become anterior NPCs in the absence of patterning factors, and also possesses the potential to differentiate along the posterior fate in the presence of patterning factors. Full size image Our success in developing the new conditions for MN derivation can be attributed to the following factors. First, the recently developed methods for rapid and highly efficient neural induction of NPCs from hESCs/hiPSCs in adherent cultures prove to be extremely beneficial for subsequent production of mature neuronal subtypes. These methods not only produce a nearly homogenous population of NPCs within a short time frame, but also can be readily modulated temporally for subsequent induction of specific neuronal lineages. Second, central to the high efficiency of MN derivation is the timing to initiate neural patterning. The differentiating cells during neural induction demonstrate remarkable sensitivity temporally to neural patterning: addition of RA at the early ( ⩽ 2 days) or the late phase (day 6) of neural induction only induces weak motoneuron fate specification (<10% efficiency), while RA addition at day 3 leads to high efficiency of MN production from hESCs (for example, 66.3% HB9 + cells from H1 hESCs). Finally, we establish new substrate conditions that lead to high rates of survival during neuronal maturation. Specifically, we identify a chemically defined mix of ECM molecules that can effectively replace the undefined Matrigel matrix. Unlike Matrigel, which fails to support survival of single differentiating cells, the combined matrix proteins of laminin, fibronectin and COLI and COLIV markedly improves single-cell survival during MN maturation (to 91%) and leads to high-yield production of MNs from hESCs (>250%). Recently, several labs used simultaneous inhibition of BMP and Activin signalling for neural induction of human pluripotent stem cells, producing high percentages of PAX6 + NPCs in 5–6 days [9] , [10] , [11] . These NPCs are thought to represent the most primitive neural–progenitor cell stage isolated to date because they show characteristics of early neuroepithelial cells of the central nervous system and can form neural rosette structures in vitro [9] . Surprisingly, in our experiments these neural progenitors are extremely refractory to patterning stimulation and only develop into a small fraction of MNs. The weak response of the NPCs indicates that these cells might be more committed along the anterior neural fate than previously recognized and thus possess declined caudalization potential. Indeed, we performed time-course analyses of expression of 20 forebrain and 19 hindbrain markers and reveal changes in cell stages during neural induction. Specifically, a majority of forebrain genes are continuously upregulated during compound C induction, while many hindbrain genes are suppressed at the end of the induction (that is, at day 6; Table 1 ). Our results are consistent with a recent report showing that prolonged dual inhibition of Activin and BMP signalling in hESCs induces differentiation of cells characteristic of the anterior neural ectoderm [11] . In addition, we demonstrate that a large population of PAX6 + /OCT-4 + cells emerges at day 3 of neural induction, when many forebrain genes exhibit relative low levels of expression (for example, WNT7B , OTX2 , NR2F1 , POU3F1/2 , EMX2 , ARX and FEZF2 ). Initiation of patterning at this more primitive stage of neural induction (at day 3) leads to a substantially higher MN differentiation efficiency (66.3% HB9 + cells versus 4.6% for day 6 for H1 hESCs; Fig. 2d ). Together, these results point to a previously unidentified primitive stage of neural progenitors that is intermediate between pluripotent hESCs and anterior NPCs ( Fig. 6b ). This population of potential primitive NPCs, which occur at day 3 of compound C induction, can be induced to become anterior NPCs with prolonged compound C treatment and also possesses the potential to differentiate posteriorly in the presence of patterning factors ( Fig. 6b ). Thus, we reveal differential cell fate decisions as a result of temporal control by patterning factors, induce high-efficiency MN differentiation from hESCs/hiPSCs via temporally modulated neural patterning and identify a potential primitive NPC stage. These findings have not been reported previously. Interestingly, the potential primitive human NPCs we have defined are reminiscent of the mouse primitive neural stem cells (pNSCs) described in earlier studies. Mouse ESCs, when cultured under defined, low-density conditions, acquire a neural–stem cell identity within 24 h [40] . These cells are multipotent, display properties that are intermediate to ESCs and forebrain NPCs [40] , and are similar to the NPCs found in the early mouse embryo (E5.5–E7.5) [40] , [41] . These embryonic cells are termed as pNSC because they are primarily neural specific but retain a certain degree of pluripotency with moderate expression of OCT-4. Unlike definitive neural stem cells, pNSCs are more primitive during neural fate specification [40] , [41] , [42] . Notably, the primitive human NPCs we have derived from hESCs exhibit similar characteristics to the mouse embryonic pNSCs. For instance, they have already begun to express high levels of neural progenitor markers but also retain some expression of pluripotency markers at the same time ( Fig. 2a and Supplementary Fig. 1 ), representing an intermediate stage between hESCs and anterior NPCs. Thus, we present evidence for a similar primitive neural–stem/progenitor–cell stage during neural specification of human pluripotent stem cells ( Fig. 6 ). In addition to its apparent values for cell-replacement therapies, our MN differentiation model is highly applicable for the study of human neural development and disease modelling. This model uses simple adherent cultures, produces abundant cells, can be readily manipulated genetically and recapitulates differentiation process in real time with high efficiency. By applying this model, we show for the first time that ISL1 acts as a key regulator of motoneuron development of hESCs. Consistent with earlier studies of mutant Isl-1 animal models, depletion of ISL1 severely impairs neuronal formation and development of mature and functional MNs from hESCs. However, ISL1 depletion, unlike ISL1 deletion and hypomorphic ISL1 mutations in mouse models, does not induce cell death or conversion to the V2a interneuron fate, implying distinct regulatory mechanisms underlying human MN development. Although a more complete understanding of the detailed mechanisms underlying ISL1’s function awaits further experimentation, these results represent a successful example of studying human MN development ‘in the dish’ and prove the effectiveness of the model for the molecular dissection of human neural specification and human MN development. Similarly, the procedure should also facilitate the application of hESCs/hiPSCs to the modelling, understanding and therapeutic strategies of human MN disorders. In sum, our findings lead to an effective new strategy for MN derivation from human pluripotent stem cells, which should facilitate the use of hESCs and hiPSCs for developmental and disease studies, drug screening and regenerative medicine. Our study also provides novel mechanistic insights into early human neural development. Cell culture H1 and H9 hESC lines (WiCell Research Institute, Madison, WI) were routinely maintained under feeder conditions or feeder-independent conditions. For feeder conditions [1] , primary mouse embryonic fibroblasts prepared from embryos of pregnant CF-1 mice (day 13.5 of gestation; Charles River) were cultured in DMEM containing 10% fetal bovine serum (Hyclone), 1 mM non-essential amino acid and penicillin/streptomycin, and mitotically inactivated by γ-irradiation. H1 and H9 cells were cultured on irradiated mouse embryonic fibroblasts in media containing DMEM/F12, 20% knockout serum replacement, 4 ng ml −1 basic fibroblast growth factor (Invitrogen), 1% non-essential amino acid, 1 mM glutamine and 0.1 mM β-mercaptoethanol. For feeder-independent conditions, hESCs were cultured on Matrigel (BD Biosciences)-coated plates in mTeSR1 medium (StemCell Technologies) or E8 medium for the support of long-term self-renewal [15] , [43] . The quality and high viability of the cells are essential for their proper responses to induction of differentiation. The MR31 and MMW2 hiPSCs were derived from human IMR90 fetal lung fibroblasts and human adult mesenchymal stem cells, respectively [10] , [35] . The ID28 hiPSCs, kindly provided by Dr Marius Wernig (Stanford University), were derived from human dermal fibroblasts using a polycistronic lentiviral vector containing the reprogramming factors, which were subsequently removed by the use of Cre recombinase [36] . The hiPSCs were cultured under the same conditions as hESCs. Reagents and antibodies ESC-qualified Matrigel, laminin-1, fibronectin, COLI and COLIV are from BD. SHH is from R&D. α-Bungarotoxin is from Molecular Probes. TTX is from Tocris Bioscience. Compound C is from EMD Biosciences. Other reagents are from Sigma. All antibodies are from commercial sources. Their sources and dilutions for western and/or immunofluorescence analyses are listed in Supplementary Table 1 . Immunofluorescence Cells were washed once with cold PBS, fixed with 4% paraformaldehyde for 10 min, permeabilized with 0.1% Triton X-100 in PBS and blocked with donkey serum. Primary antibodies in various dilutions ( Supplementary Table 1 ) were incubated with samples overnight at 4 °C, followed by fluorescein isothiocyanate (or Alexa)-conjugated secondary antibody. Nuclei were counterstained with DAPI (4',6-diamidino-2-phenylindole; Sigma). Images were collected with Axiovert 200 M microscope (Zeiss). The number of immunofluorescence-labelled cells was analysed and quantified by using Image J (NIH) and In Cell Analyzer 2000 (GE Healthcare). The synaptic structures in hESC/hiPSC-derived MNs were visualized using the Multiphoton Confocal Microscope Zeiss 710 System with the visible excitation lines at 405, 488 and 594 nm. Confocal images were collected using the Axio Observer Z1 microscope with a × 63 objective. Neural induction and MN differentiation Neural induction (that is, from hESCs/hiPSCs to NPCs) was performed as described, with some modifications [10] . Briefly, cells were gently dissociated into single-cell suspension with 1 mg ml −1 accutase for 5–7 min at 37 °C. The dissociated cells were plated at high density (10 6 cm −2 ) on Matrigel or a chemically defined matrix mix containing vitronectin, (20 μg ml −1 ) laminin (10 μg ml −1 ) and fibronectin (10 μg ml −1 ), and cultured to confluency in mTeSR1 medium or the chemically defined E8 medium. Neural induction was initiated by cultivation of cells in N2 medium containing compound C (1 μM). N2 medium is composed DMEM/F12 supplemented with 1% N2 supplement, 1 mM glutamine and 0.2% heparin. Cells were treated with compound C for 6 days. To induce neural patterning and MN differentiation, 3 days after compound C addition, RA (100 nM) was added to N2 medium (‘day 3’). Three days after RA addition, compound C was removed from N2 medium, after which both RA and SHH (100 ng ml −1 ) were included for further induction of patterning (‘day 6’). At day 9, cells were trypsinized, transferred to plates pre-coated with laminin-1, fibronectin, COLI and COLIV (LN/FN/COLI/COLIV; see below) and cultured in N2 medium containing cAMP (0.1 μM), brain-derived neurotrophic factor (10 ng ml −1 ), glial cell-derived neurotrophic factor (10 ng ml −1 ), insulin-like growth factor-1 (10 ng ml −1 ), RA (100 nM) and SHH (100 ng ml −1 ; neuronal maturation medium), and incubated until day 20. In some experiments, cells were re-plated on substrates consisting of LN/FN/COLI/COLIV at day 15 when lower cell-culture densities were favoured. To prepare ECM substrates for neuronal maturation, plates were first coated with COLI and COLIV (10 μg ml −1 ) for 1 h at room temperature and then coated with laminin (10 μg ml −1 ) and fibronectin (10 μg ml −1 ) at 4 °C overnight. To examine neuronal morphology and analyse ISL1 and HB9-positive cells counterstained with DAPI, cells were replated at lower densities after 15-day (for ISL1) and 20-day (for HB9) differentiation. Briefly, cells were gently dissociated with 1 mg ml −1 accutase for 3 min at 37 °C, followed by replating at ~10 5 cells per cm 2 on chemically defined ECM substrates containing COLI (10 μg ml −1 ), COLIV (10 μg ml −1 ), laminin (10 μg ml −1 ) and fibronectin (10 μg ml −1 ), and subsequent cultivation in neuronal maturation medium. The Rho kinase inhibitor Y-27632 (1 μM; EMD Millipore) was included in the medium to enhance cell survival. Neuronal morphology and expression of MN markers were examined 3–4 days after replating, when cell attachment and neurite extension were observed. Electrophysiological experiments Twenty days after differentiation, hESC/hiPSC-derived MNs were maintained in neuronal maturation medium. After 10 days, cells were used for whole-cell patch clamp recordings. Before recording, an individual culture slide was transferred to a submersion-type recording chamber maintained at room temperature and continuously superfused (2.0±0.25 ml min −1 ) with oxygenated (100% O 2 , pH 7.4) physiological saline. The physiological solution contained in mM: 115.0 NaCl, 2.0 KCl, 1.5 MgCl 2 , 3.0 CaCl 2 , 10.0 HEPES and 10.0 glucose (pH 7.3, 300–310 mosm). Individual neurons were visualized using an Olympus BX-51WI fixed stage microscope equipped with DODT contrast optics and a water-immersion objective (× 60, 0.9 numerical aperture, Olympus). For whole-cell current– and voltage–clamp recordings, patch pipettes had a tip resistance of 3–6 MΩ when filled with a potassium-based internal solution containing in mM: 117.0 K-gluconate, 13.0 KCl, 1.0 MgCl 2 , 0.07 CaCl 2 , 1.0 EGTA, 10.0 HEPES, 5.0 Na 2 -phosphocreatine, 2.0 Na 2 -ATP and 0.4 Na-GTP (pH 7.3, 290 mosm). Pipettes also contained 50 μM Alexa 594 (Molecular Probes) for two-photon imaging. During recordings, the pipette capacitance was neutralized and access resistance was continually monitored. In current–clamp recording mode, initial input resistance was assessed from current step injections (−20 to +120 pA, 20 pA intervals, 500 ms duration). Subsequently, action potentials were evoked by current step injections (up to 120 pA, 100–200 ms duration). Transient sodium current were evoked in voltage–clamp mode by an initial holding potential of −60 mV, then stepping the membrane potential to −100 mV (20 ms) followed by depolarizing step (−100 to +40 mV, 10 mV intervals, 50 ms duration). For imaging, individual cells were filled via recording pipette with Alexa 594 and imaged by laser excitation (820 nm) using a two-photon laser scanning microscopy system (Prairie Ultima, Prairie Technologies) coupled with a Ti-sapphire laser (MaiTai HP, Spectra Physics). After recording, stacked images were acquired (5.12 pixels per μm; 0.25–0.50 μm steps in z axis) and used to reconstruct the morphology of the cell (NIH Image J). TTX was prepared and stored as recommended by the manufacturer and subsequently diluted in physiological saline just before use. Western blotting Cells (5 × 10 6 ) were lysed directly with 200 μl laemmli sample buffer (BIO-RAD). For the analysis of other proteins, lysis buffer (0.3% Triton X-100, 20 mM Tris/HCl, pH 7.5, 0.1 mM Na 3 VO 4 , 25 mM NaF, 25 mM β-glycerophosphate, 2 mM EGTA, 2 mM EDTA, 1 mM dithiothreitol, 0.5 mM phenylmethyl sulphonyl fluoride) was used. Twenty-five microlitres of each sample were analysed by western blotting. Dilutions for various antibodies are described in Supplementary Table 1 . The blots were developed using SuperSignal West Pico Chemiluminescent Substrate (Pierce). Real-time PCR For real-time PCR experiments, total RNA were isolated with Trizol reagent (Invitrogen) according to the manufacturer’s instructions, treated with DNase I to eliminate DNA contamination and purified with RNeasy mini kit (QIAGEN). Complementary DNA was synthesized from the purified RNA using Reverse Transcription System (Promega) with random primers. Real-time PCR was performed by using SYBR Green JumpStart Taq ReadyMix (Sigma). The reaction mixture included SYBR Green mix (2 × , 12.5 μl), 10 × primer assay (2.5 μl), cDNA (1 μg) and nuclease-free water with total volume of 25 μl. The following programme was used: 95 °C for 15 min followed by 40 cycles of 94 °C for 15 s, 56 °C for 15 s and 72 °C for 34 s. Sequences of the primers are shown in Supplementary Table 2 . ACTB gene was used as internal control to equalize cDNA loading. Lentivirus production and infection For shRNA-mediated gene knockdown, pLKO vectors containing different ISL-1 shRNA sequences (Sigma-Aldrich) were used to package virus with Viralpower Lentivirus Packaging System (Invitrogen) [44] , [45] . To deliver ISL1-targeting shRNAs, hESCs were induced to undergo MN differentiation and infected with lentivirus containing ISL1 shRNAs before the induction of neuronal maturation (day 9) with a multiplicity of infection of ~100. Cells were then fixed or lysed at day 15 and day 20, respectively, and subjected to immunofluorescence and real-time PCR analyses of ISL1, TUJ1, HB9 and ChAT. The sequences for ISL1 shRNA-1 and shRNA-2 are: shRNA1: 5′-CCGGGTGACATAGATCAGCCTGCTTCTCGAGAAGCAGGCTGATCTATGTCACTTTTT-3′ and shRNA2: 5′-CCGGGCTGTTTCTATATTGGTCATTCTCGAGAATGACCAATATAGAAACAGCTTTTT-3′. For ISL1 rescue experiments, ISL1 expression vector was generated by inserting human ISL1 cDNA (OriGene SC125257) into pSin-EF2-alpha-Puro lentivector (Addgene). Lentivirus containing the ISL1 expression vector was used to infect cells before the induction of neuronal maturation, in conjunction with the ISL1 shRNA-2 lentivirus. Myotube co-culture analysis C2C12 cells were maintained in Dulbecco's Modified Eagle's Medium (DMEM) (1 g l −1 glucose) with 10% fetal bovine serum. For differentiation, cells were seeded in plates coated with 0.2% gelatin. Differentiation was induced by switching to DME containing 2% horse serum [46] . MNs derived from hESCs or hiPSCs were plated onto myotubes for 7 days, after which the neuromuscular synapses could be visualized using ChAT and BTX staining. Statistical analysis All data are presented as mean±s.d., except those for real-time PCR, in which s.e.m. was calculated. The statistical significance of the difference between the means of samples was tested by one-way analysis of variance. How to cite this article: Qu, Q. et al . High-efficiency motor neuron differentiation from human pluripotent stem cells and the function of Islet-1. Nat. Commun. 5:3449 doi: 10.1038/ncomms4449 (2014).